Rational design of a binary metal alloy for chemical vapour deposition growth of uniform single-layer graphene Controlled growth of high-quality graphene is still the bottleneck of practical applications. The widely used chemical vapour deposition process generally suffers from an uncontrollable carbon precipitation effect that leads to inhomogeneous growth and strong correlation to the growth conditions. Here we report the rational design of a binary metal alloy that effectively suppresses the carbon precipitation process and activates a self-limited growth mechanism for homogeneous monolayer graphene. As demonstrated by an Ni–Mo alloy, the designed binary alloy contains an active catalyst component for carbon source decomposition and graphene growth and a black hole counterpart for trapping the dissolved carbons and forming stable metal carbides. This type of process engineering has been used to grow strictly single-layer graphene with 100% surface coverage and excellent tolerance to variations in growth conditions. With simplicity, scalability and a very large growth window, the presented approach may facilitate graphene research and industrial applications. Graphene, a zero-bandgap semimetal with both excellent optical transparency and electrical conductivity, is a promising material for nanoscale electronics and flexible macroelectronic devices [1] , [2] . Because the various physicochemical properties of graphene are sensitive to its thickness [3] , [4] , [5] , the capability of synthesizing uniform graphene with well-controlled layer numbers has been one of the major challenges in graphene research [6] . Chemical vapour deposition (CVD) has been actively investigated since 2009 for growing graphene on catalytic metal films or foils from gaseous carbon sources at high temperatures [7] , [8] , [9] , [10] . The first CVD graphene was obtained on polycrystalline nickel (Ni) film, which has a small lattice mismatch with graphene [7] . In addition, success has been achieved recently on copper (Cu) foils. The obtained graphene films on Cu have been as large as 30 inches [11] , and 95% of the films are single-layer [9] . The ability to grow large-area, high-quality graphene and the wide accessibility of equipment make CVD growth the most competitive approach, especially for electronics applications. The general CVD process for growing graphene on metals involves the following elementary steps: adsorption and subsequent catalytic decomposition of a gaseous carbon source on metal surfaces, downward dissolution of surface carbon species into the bulk metal, upward segregation of the carbon atoms in the bulk metal onto the metal surface upon cooling and reconstruction of the surface carbon atoms into graphene [12] , [13] . The growth kinetics of graphene are further complicated by the growth pressure (typically low pressure or ambient pressure) and temperature, cooling rate, concentration of carbon sources and solubility of carbon and its temperature dependence in bulk metal [12] , [13] , [14] , [15] , [16] . All of these factors contribute to the uniformity and layer distribution of the obtained graphene films. For catalytic metals with high carbon solubility and a sharp temperature dependency, such as Ni and cobalt (Co) (~1.2 and 1.0 at.% at 1,000 o C respectively), a massive carbon species would segregate from bulk metals and precipitate on the surface during cooling [17] . This type of non-equilibrium precipitation process is believed to be the origin of inhomogeneous graphene growth, especially at the grain boundaries of polycrystalline metal films, which serve as nucleation centres for multilayer graphene growth [18] . Apparently, the cooling rates of the growth substrates strongly affect the graphene thickness and uniformity. Interestingly, the use of thin-metal films with slow cooling can suppress the excessive carbon precipitation [12] . In addition, improving the surface perfectness of the catalytic metals is effective for growing long-range ordered graphene, which has been demonstrated by recent works using heteroepitaxially deposited Ni on magnesium oxide (MgO) (111) [19] and highly crystalline Co thin film on c -plane sapphire [20] . Because Cu has a very low solubility of carbon (<0.004 at.%), the non-equilibrium precipitation process is not significant in the CVD growth of graphene [9] . As a result, graphene growth on Cu at low pressure is governed by the reconstruction process of catalytically decomposed surface carbon species, which primarily leads to single-layer graphene [13] . Recently, studies have shown that bilayer and even multilayer graphene could be obtained on copper by using a slower cooling rate and an elevated growth pressure or increased concentrations of carbon sources [14] , [21] . The dissolution of carbons into bulk metals and their subsequent non-equilibrium precipitation are the crucial steps governing the uniformity of CVD graphene. With a suitable design involving a catalytic metal system to control these processes, a facile control of graphene layer thickness could be achieved. Cu is an example of a successful attempt to grow single-layer graphene in the absence of non-equilibrium precipitation (attributable to the least carbon solubility). 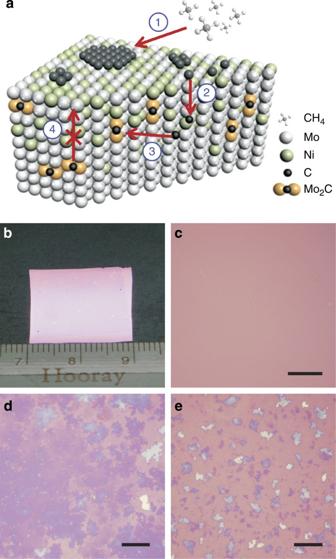Figure 1: Designed binary alloy and typical growth results on different substrates. (a) Schematic drawing of a designed binary alloy for CVD growth of single-layer graphene by suppressing carbon precipitation, which was demonstrated by an Ni–Mo model system. The numbers from 1 to 4 represent the elementary steps in the Ni–Mo-CVD process, including surface catalytic decomposition of the carbon source and reconstruction of the carbons, downward dissolution of the carbon atoms into the bulk metal, the formation of metal carbides and suppressed upward precipitation of the carbons, respectively. (b) Photograph of a 2×2 cm single-layer graphene grown on a Ni (200 nm)/Mo (25 μm) foil. (c) Optical microscope image ofb, which demonstrates the excellent uniformity of the single-layer graphene and shows that it has 100% surface coverage. Optical microscope images of CVD graphene grown on 200-nm Ni/SiO2/Si substrates at a cooling rate of (d) 20 °C min−1and (e) 4 °C min−1. The growth conditions were 1,000 °C for 5 min, ambient pressure with a gas flow of H2:CH4=16:1 sccm, and 20 °C min−1of cooling rate unless otherwise specified. The gas flow composition in (e) was H2:CH4=160:1 sccm. The graphene films were transferred onto 300-nm SiO2/Si substrates for characterization. The scale bars ofc–eare 20 μm. This study demonstrates an alternative strategy for the CVD growth of single-layer graphene using a designed binary alloy, which is schematically shown in Figure 1a . The key of our strategy is to utilize a molybdenum (Mo) component in a binary alloy to trap all of the dissolved excess carbon species in the form of molybdenum carbides, which are chemically stable throughout the high-temperature growth process [22] . Trapping all of the dissolved excess carbon species suppresses the troublesome carbon precipitation process. As a result, the growth of graphene becomes governed by a self-limited surface catalytic process, which is similar to what occurs in the Cu-CVD process. The formation of single-layer graphene is ensured even though high carbon-soluble metal components, such as Ni and Co, are used in the alloy. Figure 1: Designed binary alloy and typical growth results on different substrates. ( a ) Schematic drawing of a designed binary alloy for CVD growth of single-layer graphene by suppressing carbon precipitation, which was demonstrated by an Ni–Mo model system. The numbers from 1 to 4 represent the elementary steps in the Ni–Mo-CVD process, including surface catalytic decomposition of the carbon source and reconstruction of the carbons, downward dissolution of the carbon atoms into the bulk metal, the formation of metal carbides and suppressed upward precipitation of the carbons, respectively. ( b ) Photograph of a 2×2 cm single-layer graphene grown on a Ni (200 nm)/Mo (25 μm) foil. ( c ) Optical microscope image of b , which demonstrates the excellent uniformity of the single-layer graphene and shows that it has 100% surface coverage. Optical microscope images of CVD graphene grown on 200-nm Ni/SiO 2 /Si substrates at a cooling rate of ( d ) 20 °C min −1 and ( e ) 4 °C min −1 . The growth conditions were 1,000 °C for 5 min, ambient pressure with a gas flow of H 2 :CH 4 =16:1 sccm, and 20 °C min −1 of cooling rate unless otherwise specified. The gas flow composition in ( e ) was H 2 :CH 4 =160:1 sccm. The graphene films were transferred onto 300-nm SiO 2 /Si substrates for characterization. The scale bars of c–e are 20 μm. Full size image As exhibited by the Ni–Mo alloy, we have successfully grown strictly single-layer graphene with 100% surface coverage and excellent tolerance to variations in growth conditions. We believe that the presented approach will promote the current efforts of graphene growth and practical applications. The growth of uniform single-layer graphene and its characterization The Ni–Mo alloy was utilized as a model system to demonstrate our strategy. A Ni layer with a typical thickness of 200 nm was deposited onto an Mo foil (usually 25 μm unless specified as 200 μm) using an ultra-high-vacuum electron beam evaporator. The Ni–Mo alloy was formed by thermal annealing at 900 °C for ~20 min under the flow of argon (Ar) and hydrogen gas (H 2 ). Figure 1b shows the photographic image of an ~2×2-cm 2 graphene film that was grown on a Ni–Mo alloy surface and transferred onto a 300-nm silicon oxide/silicon (SiO 2 /Si) substrate (Methods; Supplementary Fig. S1 ). The graphene film can be clearly visualized due to its light interference [23] . An optical microscope image ( Fig. 1c ) shows the excellent uniformity and 100% surface coverage of the graphene. From the green channel contrast with respect to the underlying SiO 2 /Si substrate in the optical microscope image [12] , we confirmed that all of the graphene area had a single layer, and no multilayer graphene was observed (please also see the RGB colour image in Supplementary Fig. S2 ). Obviously, there was a marked improvement in the growth uniformity on the Ni–Mo alloy surfaces compared with the conventional Ni-CVD. Graphene films grown on polycrystalline Ni/SiO 2 /Si substrates are highly inhomogeneous (that is, characteristic of regions and islands with different layers) ( Fig. 1d ); though the uniformity can be improved by slowing down the cooling rate to 4 °C min −1 ( Fig. 1e ). Interestingly, the best reported uniformity over Ni/SiO 2 /Si substrates was only 87% of single- or bilayer graphene [12] . On the popular Cu foils, the best growth results still contain about 5% of thicker-layer graphene [9] . The graphene grown on the Ni–Mo alloy was further examined by Raman spectroscopy, transmission electron microscopy (TEM), selected-area electron diffraction and atomic force microscopy (AFM) ( Fig. 2a–c ). The Raman 2D bands, which were collected over 100 sampling points on the transferred graphene, exhibited a symmetric single Lorentzian line shape with a full width at half-maximum of <36.5 cm −1 and the intensity ratio of G to 2D bands fell into a range of 0.4–0.5, which was characteristic of single-layer graphene with high uniformity. The D to G peak intensity ratio was comparable to that reported on Ni (ref. 19 ), which indicated that the Ni–Mo system does not introduce additional defects in graphene. The single-layer feature and high crystallinity of the graphene grown on the Ni–Mo alloy were also supported by the TEM and selected-area electron diffraction studies ( Fig. 2b and inset). The preliminary high-resolution TEM data suggested that the adjacent graphene domains were connected via defective bands, where 5–7 ringed structures are resolved ( Supplementary Fig. S3 ). In addition, the AFM image shows a uniform height of ~1.1 nm, which is typical of single-layer graphene [24] , and wrinkles were also seen over the graphene surface. 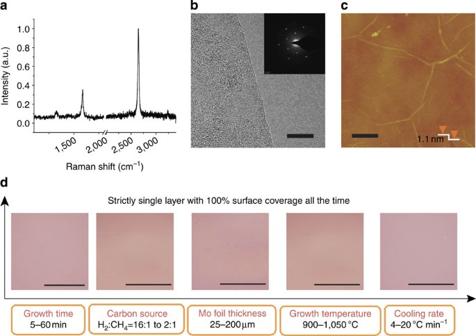Figure 2: Characterization of single-layer graphene grown on an Ni–Mo alloy and illustration of tolerance to variations in experimental conditions. (a) A typical Raman spectrum of single-layer graphene grown on an Ni–Mo alloy (excitation wavelength: 632.8 nm). (b) A TEM image and the selected-area electron diffraction pattern (inset) reveal the nice crystallinity of single-layer graphene grown on the Ni–Mo alloy. The scale bar is 10 nm. (c) An AFM image of the grown graphene shows the single-layer feature and the wrinkles. The scale bar is 500 nm. (d) Typical optical microscope images of graphene films grown on the Ni–Mo alloy under different growth conditions. The scale bar is 50 μm. All the graphenes were single layered with 100% surface coverage, which demonstrates the excellent tolerance to variations in experimental conditions. The growth conditions were 1,000oC, ambient pressure with a gas flow of H2:CH4=2:1 sccm and a cooling rate of 20 °C min−1on 200-nm Ni/25-μm Mo foil, unless otherwise specified. The other growth parameters from left to right indwere H2:CH4=16:1 sccm and 5 min growth, 30 min growth, 200-nm Ni on 200-μm Mo foil and 5 min growth, 900 °C for 10 min growth, and 4 °C min−1cooling and 5 min growth. All of the graphene samples were transferred to 300-nm SiO2/Si substrates for characterization except the TEM sample. Figure 2: Characterization of single-layer graphene grown on an Ni–Mo alloy and illustration of tolerance to variations in experimental conditions. ( a ) A typical Raman spectrum of single-layer graphene grown on an Ni–Mo alloy (excitation wavelength: 632.8 nm). ( b ) A TEM image and the selected-area electron diffraction pattern (inset) reveal the nice crystallinity of single-layer graphene grown on the Ni–Mo alloy. The scale bar is 10 nm. ( c ) An AFM image of the grown graphene shows the single-layer feature and the wrinkles. The scale bar is 500 nm. ( d ) Typical optical microscope images of graphene films grown on the Ni–Mo alloy under different growth conditions. The scale bar is 50 μm. All the graphenes were single layered with 100% surface coverage, which demonstrates the excellent tolerance to variations in experimental conditions. The growth conditions were 1,000 o C, ambient pressure with a gas flow of H 2 :CH 4 =2:1 sccm and a cooling rate of 20 °C min −1 on 200-nm Ni/25-μm Mo foil, unless otherwise specified. The other growth parameters from left to right in d were H 2 :CH 4 =16:1 sccm and 5 min growth, 30 min growth, 200-nm Ni on 200-μm Mo foil and 5 min growth, 900 °C for 10 min growth, and 4 °C min −1 cooling and 5 min growth. All of the graphene samples were transferred to 300-nm SiO 2 /Si substrates for characterization except the TEM sample. Full size image The growth window and tolerance to experimental variations The most fascinating feature of the presented CVD approach was its extremely high tolerance to variations in experimental conditions ( Fig. 2d ; Supplementary Fig. S4 and Supplementary Table S1 ). For instance, the concentration of the carbon source and the growth time dictate the total amount of carbon delivered into the reaction system. Generally, an excess carbon supply would result in the formation of thicker-layer graphene and even amorphous carbon deposits. Surprisingly, when we increased the carbon supply by ~100 times the minimum amount required to form a fully covered single-layer graphene, we still obtained uniform single-layered graphene with 100% surface coverage. No multilayer graphene spots were resolved in the highest resolution optical microscope images ( Supplementary Fig. S4 ). This was explained by the designed functionality of the Mo component in the binary alloy, which trapped and converted all of the dissolved carbon species into stable molybdenum carbides. As long as the alloy contains enough Mo to react with the dissolved carbons, a single-layer graphene would be expected. Interestingly, when the Mo foil thickness was changed from 200 to 25 μm and the Ni layer thickness was changed from 200 nm to 1,000 nm, no changes were observed in the quality of the grown graphene. The CVD growth of graphene on Cu and Ni has been shown to be sensitive to the growth temperature, which makes it difficult for thickness and uniformity to be controlled [14] , [15] . Our Ni–Mo-CVD approach was also immune to temperature variations from 900 to 1,050 °C. Below 900 °C a noticeable defect band was observed in the Raman spectrum. This was presumably due to the insufficient graphitization (data not shown), which was consistent with previous studies on Ni-CVD [15] . Moreover, the cooling rate is one of the crucial factors that significantly affect the growth quality of graphene. Slower cooling facilitates an equilibrium precipitation and leads to more uniform graphene film on Ni-CVD ( Fig. 1e ) [12] . On an Ni–Mo surface, however, variations in the cooling rate from 4 to 20 °C min −1 did not influence the growth of perfect single-layer graphene because of the complete suppression of precipitation by the formation of Mo carbides. Importantly, the carbon solubility and its temperature dependence in bulk metals are the major troublesome issues that determine the growth quality of graphene. In principle, our Ni–Mo approach ensures the growth of perfect single-layer graphene by removing the precipitation process from the growth kinetics. Our observations under various experimental conditions demonstrated that there was a very big growth window for strictly uniform single-layer graphene with the Ni–Mo-CVD approach ( Fig. 2d ). This is undoubtedly an important advantage for practical applications over the conventional CVD process. X-ray photoelectron spectroscopy (XPS) has shown direct evidence of molybdenum carbide formation in an Ni–Mo system and distinct differences in the carbon distribution in bulk Ni and Ni–Mo alloys. The characteristic C1s band that was centred at 284.6 eV on Ni–Mo alloys after CVD growth indicates the formation of high-quality graphene ( Fig. 3a ) [25] . The shoulder peak at ~283.5 eV was typical of carbidic carbon [26] , which becomes the main peak in bulk Ni–Mo alloys ( Fig. 3b ), and is achieved after removing the surface layer with argon bombardment. This suggested that the carbon species dissolved in the bulk alloy reacted with Mo to form carbides at the growth temperatures used [22] . Indeed, the formation of molybdenum carbides, predominantly Mo 2 C, was also confirmed by X-ray diffraction data ( Supplementary Fig. S5 ). A comparison of the XPS depth profile with Ni-CVD provided more decisive information to understand the single-layer-growth feature and high tolerance of Ni–Mo-CVD to variations in experimental conditions. 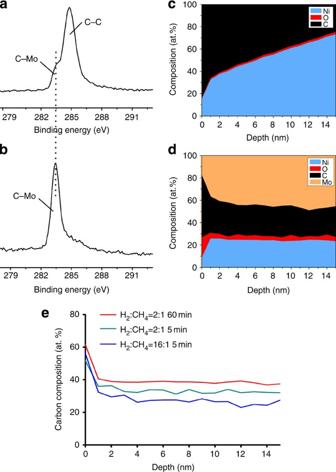Figure 3: X-ray photoelectron spectroscopic analysis of graphene on an Ni–Mo alloy surface. XPS C1s spectra of single-layer graphene grown on a Ni–Mo alloy taken at (a) the surface vicinity and (b) 15 nm downward into the bulk phase after removing the surface layer with argon bombardment. XPS composition profiles of elements along the surface normal direction on (c) 200-nm Ni/SiO2/Si and (d) 200-nm Ni/25-μm Mo foil after CVD growth (the relative composition of each element is represented by a specific colour for clarity). (e) XPS depth profiles of the carbon composition on the Ni–Mo alloy under various amounts of carbon supply. The CVD growth was performed at 1,000 °C for 5 min, with a cooling rate of 20 °C min−1and a gas flow composition of H2:CH4=16:1 sccm at ambient pressure unless otherwise specified. Figure 3c and d show the composition profiles of elements along a surface normal direction on 200-nm Ni/SiO 2 /Si and 200-nm Ni/25-μm Mo, respectively (the relative composition of each element was represented by a specific colour for clarity). On the pure Ni/SiO 2 /Si substrate, the carbon content showed a rapid monotonic decrease towards the bulk phase ( Fig. 3c ). For instance, the carbon concentrations at 2 and 15 nm from the surface were 61 and 25 at.%, respectively. This can easily be understood by taking into account the upward segregation and precipitation of carbon species from the bulk metal onto the surface during cooling. In contrast, the carbon concentration on the Ni–Mo alloy substrate remained almost unchanged in the bulk phase ( Fig. 3d ). Similar phenomena were observed even after an ~100-fold variation in the carbon supply ( Fig. 3e ). These results strongly suggest that the carbon species dissolved in the bulk phase have been converted into a non-diffusive form (that is, the stable molybdenum carbides do not allow any segregation or precipitation). Changes in the carbon supply only alter the composition of formed molybdenum carbides, and we clearly saw that larger carbon supplies correlated with increased carbide concentrations ( Fig. 3e ). Knowledge of the distribution of the elements on the topmost surface of the Ni–Mo alloy would be very interesting. Because the whole annealing, growth and cooling processes were under a reducing atmosphere with the presence of excess H 2 gas, we believe that the formation of molybdenum carbides at the topmost surface of the Ni–Mo alloy would be difficult at the experimental temperatures. The energy dispersive X-ray spectroscopy mapping showed a homogenous spatial distribution of Mo and Ni elements on the alloy surface after graphene growth ( Supplementary Fig. S6 ). Although Mo is a poor catalyst for graphene growth (data not shown), the synergistic combination of Mo and Ni works well for growing highly uniform graphene. In a conventional Ni-CVD system, the surface grain boundaries may form facile non-equilibrium precipitation paths of dissolved carbons and serve as nucleation centres, which would lead to a multilayered growth of graphene. Non-equilibrium precipitation paths, however, are effectively suppressed by carbide formation in the Ni–Mo alloy system, which allows a self-limited CVD mechanism for the growth of perfect single-layer graphene. Figure 3: X-ray photoelectron spectroscopic analysis of graphene on an Ni–Mo alloy surface. XPS C1s spectra of single-layer graphene grown on a Ni–Mo alloy taken at ( a ) the surface vicinity and ( b ) 15 nm downward into the bulk phase after removing the surface layer with argon bombardment. XPS composition profiles of elements along the surface normal direction on ( c ) 200-nm Ni/SiO 2 /Si and ( d ) 200-nm Ni/25-μm Mo foil after CVD growth (the relative composition of each element is represented by a specific colour for clarity). ( e ) XPS depth profiles of the carbon composition on the Ni–Mo alloy under various amounts of carbon supply. The CVD growth was performed at 1,000 °C for 5 min, with a cooling rate of 20 °C min −1 and a gas flow composition of H 2 :CH 4 =16:1 sccm at ambient pressure unless otherwise specified. Full size image The high quality and uniformity of single-layer graphene grown by the Ni–Mo-CVD approach have also been supported by electrical transport measurements. The dual-gated field effect transistors were fabricated on 300-nm SiO 2 /p-Si substrates using conventional electron beam lithography followed by a metal (5 nm Ti and 45 nm Au) deposition ( Fig. 4a ). A 5-nm of a high-κ dielectric material, yttrium oxide (Y 2 O 3 ) was created on the graphene film as the top-gate dielectric by evaporating the yttrium layer and performing a thermal oxidation process. 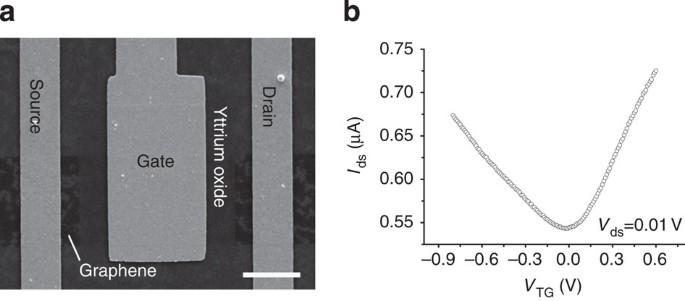Figure 4: Electrical properties of single-layer graphene grown on an Ni–Mo alloy surface. (a) A scanning electron microscopy image of the dual-gated graphene field effect transistor (FET) made on a 300-nm SiO2/p-Si substrate using electron beam lithography followed by a metal (5-nm Ti and 45-nm Au) deposition, where a Y2O3layer with a thickness of 5 nm was used as the top-gate dielectric, that was achieved by evaporating the yttrium layer and performing a thermal oxidation process. The scale bar is 3 μm. (b) The typical transfer characteristics of the fabricated graphene FET at room temperature. [27] Figure 4b demonstrates the highly reproducible transfer characteristics ( I ds - V TG ) of the field effect transistors that were measured at room temperature. The V-shaped ambipolar property is typical for single-layer graphene with a zero bandgap. The extracted electron carrier mobility was 973 cm 2 V −1 s −1 (ref. 28 ), which was consistent with the graphene grown by the conventional CVD on a Ni surface [2] , [7] . Figure 4: Electrical properties of single-layer graphene grown on an Ni–Mo alloy surface. ( a ) A scanning electron microscopy image of the dual-gated graphene field effect transistor (FET) made on a 300-nm SiO 2 /p-Si substrate using electron beam lithography followed by a metal (5-nm Ti and 45-nm Au) deposition, where a Y 2 O 3 layer with a thickness of 5 nm was used as the top-gate dielectric, that was achieved by evaporating the yttrium layer and performing a thermal oxidation process. The scale bar is 3 μm. ( b ) The typical transfer characteristics of the fabricated graphene FET at room temperature. Full size image In summary, the use of a binary alloy to suppress the carbon precipitation in the CVD process allowed us to grow strictly single-layer graphene with 100% surface coverage. This strategy is not limited to Ni–Mo alloys. Indeed, the present strategy can be extended to any alloy that contains an active catalyst component, such as Co and ruthenium (Ru), for carbon source decomposition and graphene growth as well as a black hole counterpart, such as yttrium (Y) and chromium (Cr), for trapping the dissolved bulk carbon species by converting them into stable metal carbides. Our preliminary studies have confirmed the feasibility of binary alloys using a Co-Mo alloy system in which similar highly uniform single-layer graphene was grown with 100% surface coverage ( Supplementary Fig. S7 ). The key aims of the presented approach are to effectively suppress the troublesome precipitation process of dissolved carbons and activate a self-limited growth mechanism. This type of process engineering can ensure the CVD growth of strictly uniform single-layer graphene. In addition to the extremely high tolerance of the metal alloy approach to variations in experimental conditions, the simplicity and scalability of using metal alloy foils will greatly facilitate future graphene research and industrial applications. Preparation of the Ni–Mo substrates Ni films with a thickness of 200 nm were deposited on Mo foils (25 or 200 μm) using an electron beam evaporator (ULS400, Balzers). Before deposition, the Mo foils were ultrasonicated in hydrochloric acid (HCl:H 2 O=1:1 volume) to remove the surface metal oxides. This was followed by rinses with deionized water, acetone and ethanol before being dried under a nitrogen stream. The Ni target was commercially available with a purity of >99.6 wt.% (General Research Institute for Nonferrous Metal). The 25-μm Mo foils had a purity of >99.95 wt.% and were purchased from Alfa Aesar China Co. Ltd., and the 200-μm Mo foils were purchased from Luoyang Achemetal Co. Ltd. The evaporation pressure was maintained at ~10 −4 –10 −5 Pa. CVD growth of graphene The CVD growth of graphene was carried out in a quartz tube furnace (HTF 55322C Lindberg/Blue M) under ambient pressure. The growth process primarily consisted of three steps: (1) heating the Ni–Mo substrates to 900 °C at a rate of 10–16 °C min −1 and annealing for ~20 min under the flow of Ar and H 2 for alloy formation; (2) exposure of the substrates to a carbon source at 1,000 °C for 0–60 min under the flow of methane (CH 4 ) and H 2 and (3) cooling the substrates to room temperature at a rate of 4–20 °C min −1 under Ar, H 2 and a reduced amount of CH 4 . The growth procedure is illustrated in Supplementary Figure S1 . Transferring the graphene to the target substrates The process of transferring the graphene to the target substrates involves spin coating a poly(methyl methacrylate) (PMMA) film onto the graphene-grown substrates and releasing the PMMA/graphene film by etching out Ni–Mo film in an iron (III) chloride (FeCl 3 ) aqueous solution (~1 M) for 1 h. This was followed by a rinse in HCl/ultrapure water to remove the metal ions. The PMMA layer was dissolved with hot acetone after the PMMA/graphene film was transferred onto the target substrates (for example, SiO 2 /Si). Because directly immersing the PMMA/graphene/target substrate into hot acetone often leads to the folding of graphene from its edge, we hung the sample over the boiled acetone and allowed the acetone vapour to condense onto the PMMA layer in such a way that the PMMA was gradually dissolved and flowed down with acetone droplets. Characterization Optical images were taken with an optical microscope (Olympus DX51, Olympus), and Raman spectroscopy was performed with a laser micro-Raman spectrometer (Renishaw RM1000, Renishaw, 632.8 nm excitation wavelength). The AFM images were taken with a Veeco Nanoscope IIIa (Veeco) with graphene transferred onto the 300-nm SiO 2 /Si. The TEM images were taken with a Tecnai F20 microscope and aberration-corrected, high-resolution TEM (AC-HRTEM, JEOL 2010F) with graphene samples directly transferred onto a copper grid. XPS was performed on a Kratos Analytical AXIS-Ultra using monochromatic Al Kα radiation (225 W, 15 mA, 15 kV). The scanning electron microscopy image was taken with a FEI-sFEG-XL30 microscope (FEI). The current ( I )–voltage ( V ) data were collected in the cryogenic probe station (Lakeshore) under vacuum (4×10 −3 torr). The spatial distributions of Ni and Mo on the surface were obtained by energy dispersive X-ray spectroscopy (Oxford Instrument equipped with a Hitachi S-4800 (Hitachi)). How to cite this article: Dai, B et al . Rational design of a binary metal alloy for chemical vapour deposition growth of uniform single-layer graphene. Nat. Commun. 2:522 doi: 10.1038/ncomms1539 (2011).